Sonic hedgehogcontrols growth of external genitalia by regulating cell cycle kinetics The secreted signalling molecule Sonic hedgehog ( Shh ) acts to specify positional identities and to promote cell proliferation and survival in a wide range of organ systems [1] , [2] , [3] , [4] , [5] . In the vertebrate limb and brain, for example, Shh has been proposed to integrate patterning with growth, and in both systems removal of Shh leads to altered pattern formation because of diminished proliferation of progenitor cells [6] , [7] , [8] . Although the Shh pathway can regulate expression of genes that control the cell cycle, including G1/S cyclins [4] , [5] , [6] , the cellular mechanisms by which Shh influences proliferation are not well understood. Moreover, data from multiple systems suggest varied and context-specific roles for Shh in control of the cell cycle [5] . During external genital development, a pair of swellings arises from the anterior margin of the cloaca and forms the genital tubercle, the embryonic precursor of the penis and clitoris, which then undergoes a sustained period of proximodistal outgrowth. Growth of the tubercle is coordinated with three dimensional tissue patterning and urethral tubulogenesis. Transcription of Shh begins before the initiation of genital budding in a lineage-restricted compartment of cloacal endoderm that gives rise to the urethral epithelium, and Shh expression persists through the early stages of sexual differentiation [9] , [10] . In Shh knocknot mice [11] , loss of Shh results in complete absence of external genitalia, and although mutant embryos initiate genital budding, outgrowth arrests before the formation of a genital tubercle [9] , [12] , [13] . Recent studies demonstrated that disruption of Shh signalling after initiation of the tubercle results in truncation of the phallus [14] , [15] , [16] , which raises new questions about the cellular mechanisms by which Shh integrates organ growth and pattern formation. To address the cellular and molecular mechanisms by which Shh regulates genital outgrowth, we conducted temporally controlled, tissue-specific deletions of Shh at different stages of external genital development. We find that very early, transient expression of Shh is sufficient to specify the normal spatial patterns of gene expression in the genital tubercle; however, prolonged Shh activity is required for this pattern to be expanded. Disruption of Shh signalling results in a sustained decrease in the expression of cell cycle regulatory genes that govern the G1/S transition, as well as a transient downregulation of G2/M promoting genes. Analysis of cell cycle kinetics after Shh inactivation shows that the duration of the cell cycle is increased from 8.5 to 14.4 h, and this is due to an increase in the length of G1. Consequently, fewer progenitor cells enter S-phase, which slows the rate of genital tubercle growth. We conclude that Shh controls the rate of progenitor cell proliferation, and thus progenitor pool size, by regulating the speed of the cell cycle in the genital tubercle. The finding that cell cycle regulatory genes in the limb buds and genital tubercles show similar responses to Shh inactivation suggests that regulation of cell cycle kinetics by Shh may be a fundamental aspect of appendage development. Transient Shh activity specifies pattern but growth is reduced During external genital development, Shh -expressing cells are confined to the endoderm and signal to the surrounding mesoderm and ectoderm ( Fig. 1a and study by Seifert et al . [10] ). We inactivated Shh after the initiation of genital budding using a tamoxifen-inducible cre ( Shh creERT2 ) to delete a floxed allele of Shh ( Shh C ) in Shh creERT2/C embryos [17] , [18] . To determine the time required for tamoxifen to activate cre and induce recombination, we monitored LacZ expression from the Rosa26 reporter ( R26R ) allele, which is induced in response to cre recombinase [19] . LacZ was first detectable 6 h after tamoxifen injection, with strong reporter activity observed in all sites of endogenous Shh expression 9 h after injection ( Fig. 1b ). We then identified when Shh signal transduction was terminated by monitoring expression of Ptch1 , a transcriptional readout of the Shh effector genes, Gli1 and Gli2 . Ptch1 transcripts were detected at low levels in the genitalia 12 h after tamoxifen injection, but were undetectable at 24, 48 and 72 h after injection, demonstrating complete and irreversible inactivation of Shh signalling by 24 h ( Fig. 1c ). The extent of genital tubercle outgrowth in these mutants is correlated with the duration of Shh signalling, with longer Shh exposures leading to more extensive outgrowth ( Fig. 1d ). 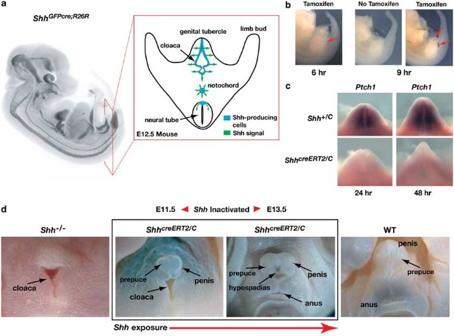Figure 1: Temporal inactivation of Shh signalling in the external genitalia. (a) Lateral view of X-gal-stainedShhGFPcre; R26Rmouse embryo at E12.5 showing position ofLacZexpression inShhGFPcredescendent cells. Image captured using optical projection tomography. Red box shows schematic of a transverse section through the external genitalia at the level of the hindlimbs and depicts the position of Shh-producing cells at the posterior end of the embryo. (b)LacZexpression (red arrows) inShhcreERT2;R26Rembryos collected 6 and 9 h after injection of pregnant dams with tamoxifen. (c) Comparison ofPtch1expression inShhcreERT2/CandShh+/Cembryos 24 and 48 h after tamoxifen injection. (d) Range of anogenital phenotypes produced by loss of Shh function at different developmental stages. All mice are males. Left panel shows complete agenesis of external genitalia and persistence of cloaca inShh−/−mutant. Middle panels show anogenital regions ofShhcreERT2/Cmice, in whichShhwas inactivated at E11.5 and E13.5 (tamoxifen injection at E10.5 and E12.5, respectively). Right panel shows normal genitalia of wild-type mouse with normal Shh activity. Figure 1: Temporal inactivation of Shh signalling in the external genitalia. ( a ) Lateral view of X-gal-stained Shh GFPcre ; R26R mouse embryo at E12.5 showing position of LacZ expression in Shh GFPcre descendent cells. Image captured using optical projection tomography. Red box shows schematic of a transverse section through the external genitalia at the level of the hindlimbs and depicts the position of Shh-producing cells at the posterior end of the embryo. ( b ) LacZ expression (red arrows) in Shh creERT2 ;R26R embryos collected 6 and 9 h after injection of pregnant dams with tamoxifen. ( c ) Comparison of Ptch1 expression in Shh creERT2/C and Shh +/C embryos 24 and 48 h after tamoxifen injection. ( d ) Range of anogenital phenotypes produced by loss of Shh function at different developmental stages. All mice are males. Left panel shows complete agenesis of external genitalia and persistence of cloaca in Shh −/− mutant. Middle panels show anogenital regions of Shh creERT2/C mice, in which Shh was inactivated at E11.5 and E13.5 (tamoxifen injection at E10.5 and E12.5, respectively). Right panel shows normal genitalia of wild-type mouse with normal Shh activity. Full size image To determine whether early removal of Shh affects the establishment of positional identity in the genital tubercle, we deleted Shh immediately after the emergence of the genital tubercle and examined the expression patterns of genes that mark specific positions of the tubercle and are required for external genital development. Wnt5a, Hoxd13 and Hoxa13 are expressed throughout the tubercle and are required for outgrowth [20] , [21] , [22] . Bmp4, Bmp7 and Msx2 mark dorsal, ventral and distal sides of the genital tubercle and regulate several aspects of genital morphogenesis [9] , [12] , [23] , [24] . Surprisingly, when the Shh pathway was inactivated as early as E11.5, although the tubercles were reduced in size, normal spatial expression of Wnt5a , Hoxd13 and Hoxa13 was maintained at E13.5 ( Fig. 2a ). Bmp4, Bmp7 and Msx2 were also maintained in appropriate spatial positions 24 and 48 h after the loss of Shh signalling, although the paired lateral domains of Bmp expression, which correspond to cells of the preputial glands in wild-type mice, were not detected in Shh conditional mutants ( Fig. 2b , Supplementary Fig. S1 ). Taken together, these results indicate that the molecular polarity of the tubercle is maintained in the absence of Shh signalling, demonstrating that only transient exposure to Shh is required to establish the normal spatial patterns of gene expression. 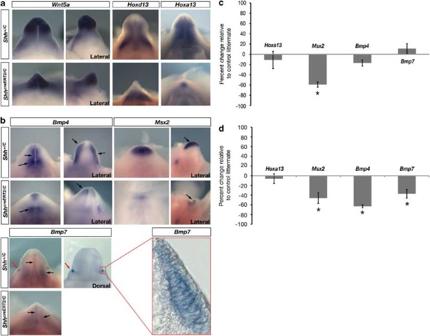Figure 2: Early and transient Shh expression is sufficient for pattern specification in the genital tubercle. (a,b) Whole mountin situhybridizations showing gene expression patterns in genital tubercles ofShhcreERT2/Cand controlShh+/cmice. Genital tubercles are shown in ventral view, except where indicated.Shhwas inactivated by tamoxifen injection at E10.5, immediately after initiation of tubercle outgrowth, and embryos were collected at E12.5 (Bmp4,andMsx2) or E13.5 (Wnt5a, Hoxd13, Hoxa13, Bmp7). Genital tubercles are reduced in size but show normal spatial expression patterns except for absence ofBmp7expression in preputial glands (red arrow inb). Black arrows mark regionalized gene expression domains. Enlargement (red box) showsBmp7-expressing preputial gland cells in control littermate. (c,d) qRT–PCR data for genes shown in (a) and (b). Embryos were injected with tamoxifen at E10.5 and collected at E12.5 (c), and injected at E11.5 and collected at E13.5 (d). Transcript levels expressed as percentage relative to control littermates, withn=3 for each data point. Error bars show ± s.e.m. and asterisks denote significant differences in (c)Msx2(P=0.009) and (d)Msx2(P=0.013),Bmp4(P=0.002) andBmp7(P=0.010). Figure 2: Early and transient Shh expression is sufficient for pattern specification in the genital tubercle. ( a , b ) Whole mount in situ hybridizations showing gene expression patterns in genital tubercles of Shh creERT2/C and control Shh +/c mice. Genital tubercles are shown in ventral view, except where indicated. Shh was inactivated by tamoxifen injection at E10.5, immediately after initiation of tubercle outgrowth, and embryos were collected at E12.5 ( Bmp4, and Msx2 ) or E13.5 ( Wnt5a, Hoxd13, Hoxa13, Bmp7 ). Genital tubercles are reduced in size but show normal spatial expression patterns except for absence of Bmp7 expression in preputial glands (red arrow in b ). Black arrows mark regionalized gene expression domains. Enlargement (red box) shows Bmp7 -expressing preputial gland cells in control littermate. ( c , d ) qRT–PCR data for genes shown in ( a ) and ( b ). Embryos were injected with tamoxifen at E10.5 and collected at E12.5 ( c ), and injected at E11.5 and collected at E13.5 ( d ). Transcript levels expressed as percentage relative to control littermates, with n =3 for each data point. Error bars show ± s.e.m. and asterisks denote significant differences in ( c ) Msx2 ( P =0.009) and ( d ) Msx2 ( P =0.013), Bmp4 ( P =0.002) and Bmp7 ( P =0.010). Full size image Although spatial domains of gene expression appeared normal in Shh creERT2/C mutant embryos, patterning defects could result from diminished levels of transcriptional activity. We therefore deleted Shh and quantified gene expression levels 48 h after tamoxifen injection. When Shh was inactivated by an E10.5 injection, only Msx2 showed a significant decrease ( Fig. 2c ). This was initially surprising, given that Msx2 is regulated by Bmp4 and Bmp7 in limb buds, however, in the early genital tubercle Msx2 and Bmp4/7 show little (if any) overlap, suggesting the presence of other Shh-dependent regulators of Msx2 at this stage. Deletion of Shh by an E11.5 injection resulted in small but significant decrease in Msx2 as well as Bmp4 and Bmp7 ( Fig. 2b,d and Supplementary Fig. S1 ). The quantitative reduction in Bmp4 and Bmp7 levels at E13.5 most likely reflects downregulation in two areas that normally express Shh ; mutants show decreased signal in and around the urethral plate ( Fig. 2b and Supplementary Fig. S1 ), and absence of signal where the preputial glands normally form ( Fig. 2b ). Loss of gene expression in the preputial glands correlated with ventral hypoplasia of the prepuce, which normally surrounds the tubercle, suggesting that preputial development might be partly governed by Shh. Collectively, the spatial expression patterns observed by in situ hybridization and the quantitative levels of expression detected by quantitative reverse transcription–polymerase chain reaction (qRT–PCR) suggest that transient Shh activity at the initiation of outgrowth is sufficient for the normal pattern specification in the genital tubercle, but that sustained Shh activity is required for transcription to be maintained at appropriate levels. Shh controls cell number and expression of cell cycle genes Once a molecular pre-pattern has been established in a developing organ, elaboration of the pattern requires extensive growth. To dissect the role of Shh in the expansion of genital tubercle progenitor cells, we quantified genital tubercle volume and total cell number in Shh creERT2/C mutant and control embryos ( Fig. 3a–f ). Twenty-four hours after inactivation of Shh signalling, genital tubercle volume and total cell number were decreased by ∼ 75% ( t (4) =3.64, P =0.01 and t (4) =2.92, P =0.02 respectively; Fig. 3b–e ). Neither cell death nor cell density differed significantly (for density, t (4) =1.33, P =0.12; Fig. 3f and Supplementary Fig. S2 ), indicating that the reduction in progenitor cell number was not due to dying cells. To test the hypothesis that the growth deficiency reflected a disruption of cell proliferation, we first searched for Shh target genes that could mediate its mitogenic effects. The transcription factors Foxf1 and Foxf2 , which have been implicated in Shh-mediated control of the cell cycle [25] , [26] , were downregulated within 24 h of Shh inactivation ( Supplementary Fig. S3 ). We next used the quantitative RT 2 –PCR Profiler Array to monitor the response of 84 genes involved in cell cycle regulation, and compared Shh creERT2/C mutant and control genitalia at different time points after inactivation of Shh ( Fig. 4a,b ). Examination of cell cycle genes 24 h after tamoxifen injection revealed significant reductions in the levels of cell cycle control genes that control both the G1/S transition ( Cyclin E1, Dp1 ) and G2/M-phase progression ( Cyclin B1 , Cdc25a ; Fig. 4a,b ). Cyclin E1 , Dp1 and the Dp binding partner E2f1 remained significantly reduced for at least 24 h after Shh inactivation, suggesting a sustained disruption in G1 progression ( Fig. 4a,b ). Myc levels also decreased (see below and Fig. 4c ) but three Cdk inhibitors, Cdkn1a, Cdkn1b and Cdkn2a , did not change significantly ( P =0.64, 0.959 and 0.492, respectively). We also observed a significant decrease in the S-phase promoting gene Cyclin A1 and a small but significant decrease in the helicase components Mcm2 and Mcm3 , which are involved in DNA replication ( Fig. 4a,b ). These results show that loss of Shh causes a transient downregulation of G2/M promoting genes and a sustained decrease in the expression of genes that govern the G1/S transition. Our discovery that Shh regulates expression of Myc , Rb1 , Dp1 and E2f1 suggests a novel mechanism by which Shh can exercise fine-scale control of cyclin levels through control of cyclin modifiers. 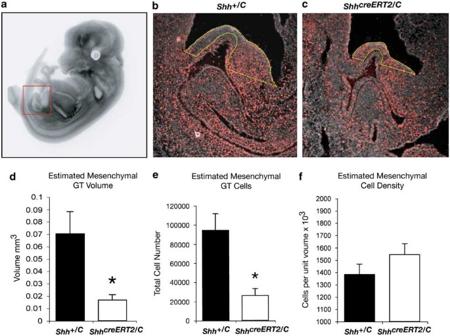Figure 3: Stereological estimates reveal decreased cell number in Shh-depleted genitalia. (a–c) Genital tubercles ofShhcreERT2/Cand controlShh+/cembryos are shown at E12.5. Pregnant females were injected with tamoxifen at E10.5 and with BrdU 44 h later. (a) Lateral view of E12.5ShhGFPcre;R26Rembryo stained with X-Gal to showShh-expressing cells10. Red box marks region of genital tubercle (gt) and underlying cloacal endoderm shown in (b) and (c). (b,c) ControlShh+/C(b) andShhcreERT2/C(c) embryos at ×10 magnification showing BrdU-labelled cells (red). (d–f) Estimates of volume (d) total mesenchymal cell number (e) and cell density (f) inShhcreERT2/C(white bars;n=3) and controlShh+/c(black bars;n=3) embryos. Data represented as means with ± s.e.m. *P<0.05. Figure 3: Stereological estimates reveal decreased cell number in Shh-depleted genitalia. ( a – c ) Genital tubercles of Shh creERT2/C and control Shh +/c embryos are shown at E12.5. Pregnant females were injected with tamoxifen at E10.5 and with BrdU 44 h later. ( a ) Lateral view of E12.5 Shh GFPcre ;R26R embryo stained with X-Gal to show Shh -expressing cells [10] . Red box marks region of genital tubercle (gt) and underlying cloacal endoderm shown in ( b ) and ( c ). ( b , c ) Control Shh +/C ( b ) and Shh creERT2/C ( c ) embryos at ×10 magnification showing BrdU-labelled cells (red). ( d – f ) Estimates of volume ( d ) total mesenchymal cell number ( e ) and cell density ( f ) in Shh creERT2/C (white bars; n =3) and control Shh +/c (black bars; n =3) embryos. Data represented as means with ± s.e.m. * P <0.05. 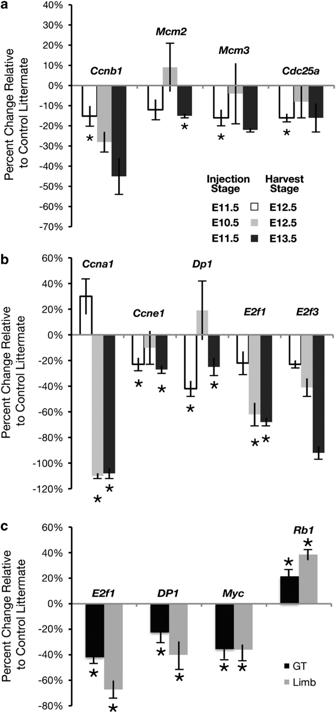Figure 4: Shh inactivation alters cell cycle gene expression in genital tubercles and limb buds. (a,b) Quantitative comparison of transcript levels inShhcreERT2/CandShh+/cembryos assayed at three time points (indicated in key) using the RT2-Profiler PCR Array (SABiosciences). Tamoxifen injections were administered at E10.5 and E11.5. Changes in transcript level are expressed as percent change relative to control embryos for G/S-phase cell cycle genes (a) and S- and G2/M-phase genes (b). Error bars show ± s.e.m.,n= 3 and asterisks denote significant differences for E11.5 injection/E12.5 collection (Cyclin E1, P=0.030;Dp1, P=0.055;Cyclin B1, P=0.019;Cdc25a, P=0.034;Mcm3, P=0.031), E10.5 injection/E12.5 collection (Cyclin A1, P=0.011;E2f1, P=0.013), E11.5 injection/E13.5 collection (Cyclin A1, P=0.0004;Cyclin E1, P=0.027;Dp1, P=0.033;E2f1, P=0.010;Mcm2, P=0.052). (c) Graph shows comparison of transcript levels in limb buds (grey bars) and genital tubercles (black bars) ofShhcreERT2/Crelative toShh+/Cembryos. Tamoxifen injections were administered at E10.5 and embryos were collected for qRT–PCR at E12.5. Changes in transcript level are expressed as percent change relative to control embryos. Error bars show ± s.e.m.,n= 3 and asterisks denote significant differences inE2f1(GT,P=0.010; limb,P=0.008),Dp1(GT,P=0.012; limb,P=0.026),Myc(GT,P=0.034; limb,P=0.039) andRb1(GT,P=0.040; limb,P=0.040). Full size image Figure 4: Shh inactivation alters cell cycle gene expression in genital tubercles and limb buds. ( a , b ) Quantitative comparison of transcript levels in Shh creERT2/C and Shh +/c embryos assayed at three time points (indicated in key) using the RT 2 -Profiler PCR Array (SABiosciences). Tamoxifen injections were administered at E10.5 and E11.5. Changes in transcript level are expressed as percent change relative to control embryos for G/S-phase cell cycle genes ( a ) and S- and G2/M-phase genes ( b ). Error bars show ± s.e.m., n = 3 and asterisks denote significant differences for E11.5 injection/E12.5 collection ( Cyclin E1, P =0.030; Dp1, P =0.055; Cyclin B1, P =0.019; Cdc25a, P =0.034; Mcm3, P =0.031), E10.5 injection/E12.5 collection ( Cyclin A1, P =0.011; E2f1, P =0.013), E11.5 injection/E13.5 collection ( Cyclin A1, P =0.0004; Cyclin E1, P =0.027; Dp1, P =0.033; E2f1, P =0.010; Mcm2, P =0.052). ( c ) Graph shows comparison of transcript levels in limb buds (grey bars) and genital tubercles (black bars) of Shh creERT2/C relative to Shh +/C embryos. Tamoxifen injections were administered at E10.5 and embryos were collected for qRT–PCR at E12.5. Changes in transcript level are expressed as percent change relative to control embryos. Error bars show ± s.e.m., n = 3 and asterisks denote significant differences in E2f1 (GT, P =0.010; limb, P =0.008), Dp1 (GT, P =0.012; limb, P =0.026), Myc (GT, P =0.034; limb, P =0.039) and Rb1 (GT, P =0.040; limb, P =0.040). Full size image Cell cycle gene regulation is conserved in limbs and genitalia Cyclin D1, which has been reported to be a target of Shh signalling in other contexts [6] , [27] , [28] , showed no significant differences between Shh creERT2/C mutant and control genitalia by two independent quantitative analyses (qRT–PCR, P =0.743;. RT 2 Profiler Array, P =0.251). This led us to investigate whether the Shh pathway acts on different cell cycle regulators in different tissues. We compared E12.5 limb buds and genital tubercles in which Shh had been inactivated at E11.5 (by tamoxifen injection 24 h earlier), when Shh is expressed in both structures. qRT–PCR analysis showed that, as in the genital tubercle, mutant and control limb buds at E12.5 showed no significant difference in Cyclin D1 expression levels ( P =0.788). However, the limb buds and genital tubercles undergo significant decreases in E2f1, Dp1 and Myc expression, and significant increases in expression of Rb1 , a negative regulator of S-phase entry ( Fig. 4c ). Given that Rb1 binds and inactivates E2f1 (study by Rubin et al . [29] ), the consequence of decreased levels of E2f1 and increased levels of Rb1 would be an even further reduction of E2f1 activity during the G1–S transition, both in the genital tubercle and limb bud. These findings show that Shh can control the same cell cycle regulators in different tissues, suggesting that conserved mechanisms may mediate the ability of Shh to regulate outgrowth of different types of appendages. Cell cycle kinetics are disrupted by Shh inactivation The finding that Shh controls quantitative levels of expression of multiple cell cycle regulators raised the possibility that the growth deficiency of Shh creERT2/C genitalia could be caused by disruption of the cell cycle. Given that genital outgrowth slows but does not arrest after Shh inactivation, we tested the hypothesis that Shh may regulate the rate of genital outgrowth by regulating the kinetics of the cell cycle [8] . Cell proliferation kinetics were examined quantitatively by calculating the proportion of cells in different phases of the cell cycle in the genitalia of Shh creERT2/C embryos. To label cells in S-phase, bromodeoxyuridine (BrdU) was injected 20 h after inactivation of the Shh pathway and embryos were allowed to develop in utero for 4 h to allow sufficient time for BrdU-labelled cells to transition from S-phase to G2/M-phase. Embryos were then harvested and labelled with antibodies against BrdU and phosphorylated Histone H3 (PHH3), a marker for cells in G2/M-phase [30] . We calculated the proportion of mesenchymal cells that were labelled with BrdU alone (S-phase), PHH3 alone (G2/M-phase), double labelled with BrdU and PHH3 (S-phase cells that had moved into G2/M-phase within 4 h) or were unlabelled (G0/G1) ( Fig. 5 ; see Methods section). An analysis of variance revealed differences in the proportion of cells in S-phase, G2/M-phase and G0/G1 in Shh creERT2/C mutant versus Shh +/C littermates that approached significance (F (2,8) =4; P =0.06). Planned comparisons of the proportion of cells in S-phase, G2/M-phase and G0/G1 phase indicated that Shh creERT2/C mutant animals ( n =3) had an 8% decrease in S-phase cells ( P =0.03) and a 7% increase in G0/G1-phase cells ( P =0.05) relative to Shh +/C littermates ( n =3; Fig. 5a ). The observation that Shh creERT2/C mutants exhibit a reduction in the number of cells in S-phase and a concomitant increase in the proportion of cells in G0/G1 is consistent with our finding that genes regulating the G1/S transition are reduced, and suggests that progression through G1 or the G1/S checkpoint is disrupted when Shh is removed. 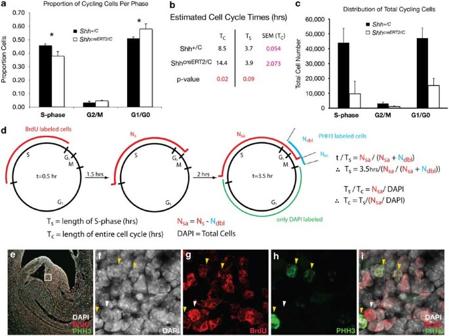Figure 5: Shh controls growth of the genital tubercle by regulating cell cycle kinetics. (a) Proportion of cells in each phase of the cell cycle. Labelling scheme groups G2 and M. Error bars show s.e.m.,n= 3, *P<0.05. (b) Estimated cell cycle times forShhcreERT2/C(mutant) andShh+/c(control) embryos. Means are shown for mutant and control embryos and s.e. of the mean is provided for Tc. (c) Total cell number calculated for each phase of the cell cycle at E12.5. Error bars show s.e.m.,n= 3. (d) Summary of cell labelling scheme used to determine lengths of S-phase (Ts) and total cell cycle (Tc). The red arcs refer to cell population labelled with BrdU, the blue arc refers to cell population labelled with phosphohistone-H3, and green arc refers to cell population labelled with only DAPI (arc lengths not to scale). (e) Sagittal section through genital tubercle ofShhC/+embryo at E12.5 shown at ×10 magnification. White box depicts area of counting frame used for cell counts. (f–i) High magnification (×145), single channel (f–h) and merged (i) exposures of boxed area in (e) showing cells labelled with DAPI (white, panelf) BrdU (red, panelg), phosphohistone-H3 (green, panelh). Yellow arrowheads mark examples of cells positive for both PHH3 and BrdU, and the white arrowhead marks a cell positive for BrdU but negative for PHH3. Figure 5: Shh controls growth of the genital tubercle by regulating cell cycle kinetics. ( a ) Proportion of cells in each phase of the cell cycle. Labelling scheme groups G2 and M. Error bars show s.e.m., n = 3, * P <0.05. ( b ) Estimated cell cycle times for Shh creERT2/C (mutant) and Shh +/c (control) embryos. Means are shown for mutant and control embryos and s.e. of the mean is provided for T c . ( c ) Total cell number calculated for each phase of the cell cycle at E12.5. Error bars show s.e.m., n = 3. ( d ) Summary of cell labelling scheme used to determine lengths of S-phase (T s ) and total cell cycle (T c ). The red arcs refer to cell population labelled with BrdU, the blue arc refers to cell population labelled with phosphohistone-H3, and green arc refers to cell population labelled with only DAPI (arc lengths not to scale). ( e ) Sagittal section through genital tubercle of Shh C/+ embryo at E12.5 shown at ×10 magnification. White box depicts area of counting frame used for cell counts. ( f – i ) High magnification (×145), single channel ( f – h ) and merged ( i ) exposures of boxed area in ( e ) showing cells labelled with DAPI (white, panel f ) BrdU (red, panel g ), phosphohistone-H3 (green, panel h ). Yellow arrowheads mark examples of cells positive for both PHH3 and BrdU, and the white arrowhead marks a cell positive for BrdU but negative for PHH3. Full size image A longer G1 phase underlies the growth defect in Shh mutants How could these relatively small proportional shifts in cell cycle phase lead to the large growth differences that result from deletion of Shh? If Shh is involved in regulating G1/S and G2/M transitions, then one possibility is that loss of Shh signalling induces cells to arrest at specific cycle checkpoints, thereby arresting proliferation or inducing apoptosis; however, such changes did not occur after deletion of Shh ( Fig. 1d and Supplementary Fig. S2 ). Alternatively, inactivation of Shh could decrease the rate of progression through G1, which would be reflected by increased cycle length. To calculate cell cycle kinetics of progenitor cells in the developing genital tubercle mesenchyme, we applied the principles developed by Nowakowski et al . [31] for quantification of cell cycle length. The relative lengths of S-phase (T S ) and the entire cell cycle (T c ) were determined for both Shh creERT2/C ( n =3) and wild-type littermates ( n =3) by measuring the proportions of cells in S-phase (BrdU/4,6-diamidino-2-phenylindole (DAPI) positive), S-phase cells that have cycled through G2/M (BrdU/PHH3/DAPI positive) and unlabelled cells (DAPI positive; see formulas in Fig. 5d and labelled cells in Fig. 5e–i ). Inactivation of Shh signalling at E11.5 resulted in lengthening of the entire cell cycle (T c ) from 8.5 to 14.4 h ( t (4) =2.83; P =0.024) ( Fig. 5b ). BrdU analysis revealed a greater proportion of unlabelled cells in Shh creERT2/C mutants ( t (4) =1.62; P =0.09), suggesting that this lengthening is not a result of altered S-phase duration but more likely reflects a delay in G1 or the G1/S checkpoint ( Fig. 5b ). Such a marked increase in cell cycle duration would be expected to reduce the total cell number, which may account for the ∼ 75% reduction of tubercle volume in Shh creERT2/C mutants. Indeed, when the proportion of cells in each phase of the cell cycle is weighed against total cell number, the data show that the loss of Shh signalling decreases the cycling cell population by ∼ 73% ( Fig. 5c ). Thus, loss of Shh activity lengthens the time that cells spend in G1/G0, thereby reducing the number of cells in S-phase, which, in turn, feeds fewer cells into G2/M-phase and, ultimately, back into the cell cycle ( Fig. 6 ). Taken together, these data indicate that Shh controls the rate of progenitor cell proliferation, and thus progenitor pool size, by regulating the speed of the cell cycle. This highlights a novel mechanism for Shh-mediated control of organ growth. 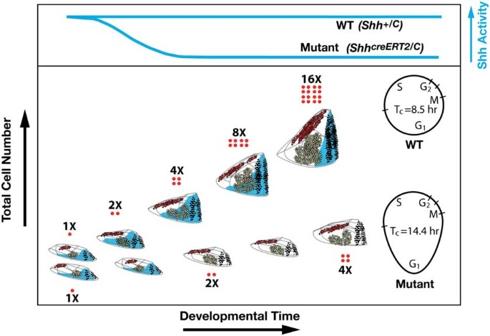Figure 6: A model forShh-mediated integration of growth and patterning. Shh activity in wild-type (WT) andShhcreERT2/C(mutant) genital tubercles is shown in top panel, and is based on analysis ofPtch1expression (seeFig. 1c). During outgrowth of the genital tubercle, cell populations (red, tan, black coloured circles) defined by regionalized gene expression are exposed to secreted Shh (blue shaded areas). In wild-type genitalia, these cells divide approximately every 8.5 h and, as these progenitor pools double in number, this expands gene expression patterns. Following loss of Shh activity in mutant genitalia, cells continue to divide but cell cycle length increases to 14.4 h. This leads to a reduction in both the doubling rate of progenitor pools and the overall size of the genital tubercle. The general molecular pattern of the mutant tubercle is retained. Large red circles above and below tubercles represent the doubling time of all cells in the genital tubercle. Tc, total cell cycle time. Figure 6: A model for Shh -mediated integration of growth and patterning. Shh activity in wild-type (WT) and Shh creERT2/C (mutant) genital tubercles is shown in top panel, and is based on analysis of Ptch1 expression (see Fig. 1c ). During outgrowth of the genital tubercle, cell populations (red, tan, black coloured circles) defined by regionalized gene expression are exposed to secreted Shh (blue shaded areas). In wild-type genitalia, these cells divide approximately every 8.5 h and, as these progenitor pools double in number, this expands gene expression patterns. Following loss of Shh activity in mutant genitalia, cells continue to divide but cell cycle length increases to 14.4 h. This leads to a reduction in both the doubling rate of progenitor pools and the overall size of the genital tubercle. The general molecular pattern of the mutant tubercle is retained. Large red circles above and below tubercles represent the doubling time of all cells in the genital tubercle. T c , total cell cycle time. Full size image These studies demonstrate that transcriptional levels of genes that control the G1/S transition are quantitatively regulated by the Shh pathway during external genital and limb outgrowth. This extends previous in vitro studies that showed that Shh and its downstream effectors can interact with specific cell cycle proteins to drive both growth phases of the cell cycle [4] , [5] , [6] , [8] , [32] . Our finding that Shh activity determines the level of Dp1 and its E2f binding partners, which are activators of Cyclin E and A1 , may account for the reduced Cyclin levels in Shh mutant embryos. Cyclin E and A1 expression may be further refined by Shh through the increased negative regulation of Rb1 , which limits E2f1 activity. Although hedgehog gain-of-function studies have suggested a role for Cyclin D1 in Shh-mediated control of cell proliferation, our quantitative analysis showed minimal changes in Cyclin D1 levels in mouse limbs and genitalia after the loss of Shh, which is consistent with results from the chick limb [6] . Taken together, these data reveal new molecular mechanisms for Shh-mediated regulation of cell cycle length, specifically the duration of G1 and the G1/S transition, and highlight how subtle changes in the kinetics of the cell cycle are amplified over developmental time to alter morphological pattern. On the basis of these results, we suggest that after the early pattern is specified in the genital tubercle, Shh promotes its elaboration and growth by regulating the length of the cell cycle ( Fig. 6 ). The control mechanism identified here may also operate in other signalling pathways and has implications for other developing organs. In the limb, for example, two recent studies reported that Shh specifies digit identity at early stages and that sustained expression is required for proliferation of progenitor cells and normal elaboration of skeletal pattern [6] , [7] . Both studies reported changes in the proportion of cells in different phases of the cell cycle, although how such changes can lead to a reduction of organ growth is not well understood at the cellular level. In light of our finding that Shh signalling determines the length of specific cell cycle phases, and that Shh regulates the same cell cycle control genes in the genital tubercle and limb bud, one possibility is that the loss of digits and the proximodistal truncations associated with reduced Shh activity in the limb may be caused by temporal changes in cell cycle kinetics, similar to those observed in the genitalia. Factors that alter cell cycle rates during the development can influence the morphology and size of an organ, and this may reflect the extent to which the early pattern has been amplified during growth [33] . Shh-mediated modulation of cell cycle duration may also underlie heterochronic changes during morphological evolution. For example, temporal truncation of Shh expression in the limb bud is associated with decreased proliferation and reduction of digit number in skinks [34] . Our results predict that such a reduction of Shh activity would lengthen cell cycle duration and thereby decrease the progenitor cell population in the limb. Similarly, the ability of hedgehog to alter cell cycle length may influence the rate of tumour growth in hedgehog pathway-mediated cancers [35] . Thus, these findings highlight the potential for modulators of cell cycle length to result in phenotypic changes in development, disease and evolution. Animals The Shh GFPcre , Shh creERT2 , Shh C and R26R alleles have been described elsewhere [17] , [18] , [19] . Tamoxifen (3 mg dissolved in corn oil) was administered to pregnant females at E10.5, E11.5 and E12.5 to induce cre-mediated deletion of Shh C . BrdU (100 mg per kg) was injected 44 h after tamoxifen to label cells in the S-phase of mitosis, and pups were collected 4 h later for analysis of cell cycle kinetics. All animal experiments were performed in accordance with institutional guidelines. Immunohistochemistry Tissue was incubated in rat anti-BrdU (1:500; Accurate) and mouse anti-phosphorylated Histone-H3 (1:500; Upstate) overnight at 4 °C and then in the minimally cross-reactive secondary donkey anti-rat Cy3 and donkey anti-mouse Cy5 (1:500, Jackson Immunoresearch) antibodies overnight at 4 °C. The tissue was washed repeatedly between steps with tris-buffered saline. Live embryos were immersed in Lysotracker Red (1:5,000; Molecular Probes) at 37 °C for 30 min to label regions of cell death, then washed in phosphate-buffered saline and dehydrated in methanol for imaging. In situ hybridization Whole mount in situ hybridization was conducted according to published methods [9] using digoxigenin-lablelled riboprobes for Shh (kindly provided by A. McMahon) , Wnt5a (A. McMahon), Ptch1 (M. Scott) Hoxd13 (D. Duboule) , Hoxa13 (S. Stadler), Bmp4 (B. Hogan) , Bmp7 (B. Hogan), Msx2 (R. Hill), FoxF1 (P. Carlsson) and FoxF2 (P. Carlsson). Quantitative RT–PCR Shh creERT2/C and control ( Shh +/c ) mice were collected from the same litters of tamoxifen-treated mothers. Genital tubercles were dissected from stage-matched embryos and were pooled according to genotype for each litter collected. RNA was extracted using Trizol. After treatment with RNase-free DNase I (Ambion), three pooled samples for each genotype were purified using the RNeasy Mini kit (Qiagen). RNA quantity and purity were determined using a NanoDrop ND-1000, and RNA integrity was assessed by determining the RNA integrity number and 28S/18S ratio using a Bioanalyzer 2100 (Agilent Technologies). A quantity of 500 ng of high-quality RNA (260/280 ratios slightly higher than 2.0 and 260/230 ratios higher than 1.7, RIN>8.0) for each pooled sample was converted into cDNA using the RT 2 First Strand cDNA Kit (SABiosciences). All qPCR reactions use the RT 2 SYBR Green qPCR Master Mix (SABiosciences). Cell cycle gene expression was determined using Cell Cycle PCR Array (PAMM-020, SABiosciences) and the My iQ5 system (Bio-Rad) according to the manufacturer's protocol. All significant changes in gene expression levels are reported in the article; the complete list of genes assayed on the array can be found at the manufacturer's website ( http://www.sabioscience.com/rt_pcr_product/HTML/PAMM-020A.html ). For patterning genes and additional cell cycle genes, expression was detected using the My iQ5 QPCR system (Bio-Rad) with Actb and Gapdh [36] as controls. Primers not previously published were designed using Beacon Designer Software (except for Actb, which was purchased from http://www.realtimeprimers.com ). The qRT–PCR primers designed for this study are listed in Table 1 . Table 1  qRT–PCR primer sequences. Full size table Stereological estimates of total cell numbers Total (DAPI-labelled), S-phase (BrdU-labelled), S- and G2/M-transition phase (BrdU/PHH3) and G2/M-phase (PHH3) cells were estimated stereologically using the optical fractionator method by counting target cells on every 12th midsagittal section ( ∼ 6 sections through the entire mediolateral axis of mesenchyme in both Shh creERT2/C mutants and control littermates), following published methods for counting cells through irregularly shaped structures, such as brain regions or kidneys [37] , [38] . Briefly, cells of interest were counted on images acquired using a ×10 objective, N.A. 0.3 on an AxioObserver Microscope and AxioVision Software (version 4.1; Zeiss). Section thickness was confirmed to be ∼ 12 μm by focusing through the sample. Cells that fell within the 45×45 μm counting frame (in a sampling grid of 235×235 μm) were used in the analyses. To estimate total mesenchymal volume, the area of mesenchyme on each section was traced and quantified using AxioVision software and the total volume of the structure was estimated using Cavalieri's principle [37] . Densities were determined by dividing the number of cells in the region of interest by the area in which the cells were counted (that is, 45×45 μm). Proportions of cells were calculated by counting total cells (DAPI-labelled) and S-phase cells (BrdU-labelled) in five separate counting frames per section, and G2/M-transition phase (BrdU/PHH3) and G2/M-phase (PHH3) cells were counted on the entire section. This was performed to avoid subsampling errors due to the low number of PHH3-positive cells per section. Cell cycle kinetics Females were injected with tamoxifen and BrdU as described in the text. S-phase and total cell cycle length were calculated according to equations in Figure 5 . BrdU labels cells approximately 30 min after injection [39] , [40] and is metabolized in approximately 2 h, [31] , [39] . Given that S-phase in both mouse and chick mesenchyme (paraxial and lateral plate) in vivo is at least 3 h [41] , [42] , a 4-h interval between injection and collection was chosen to allow BrdU-labelled mesenchymal cells to transition from S-phase to G2/M-phase. Although this may result in slight under-representation of cells that transitioned from G1- to S-phase after BrdU metabolism, and cells in late S-phase would be BrdU positive in early G2, on the basis of the relative nature of the proportion calculations, the percentages reported for each phase are accurate using this labelling scheme. Statistical analysis All group differences in our dependent variables were revealed using Student's t -tests (one dependent variable between groups) or analysis of variances (more than one dependent variable between groups) and explored using Newman–Kewls post hoc tests. α -Levels were set at 0.05. Volumetric measures Tubercle mesenchyme volume differences between Shh creERT2/C and wild-type littermates were determined using Cavalieri's principle [37] . Total cell numbers were estimated for G1/G0 (DAPI positive), S-Phase (BrdU positive) and G2/M-phase (BrdU/PHH3 positive cells) using the optical fractionator principle on every 12th section through the structure ( ∼ 6 sections per animal) [37] . Proportions and densities of cells were also calculated in different phases of the cell cycle. How to cite this article: Seifert, A.W. et al . Sonic hedgehog controls growth of external genitalia by regulating cell cycle kinetics. Nat. Commun. 1:23 doi: 10.1038/1020 (2010).